A continuous metal-insulator transition driven by spin correlations 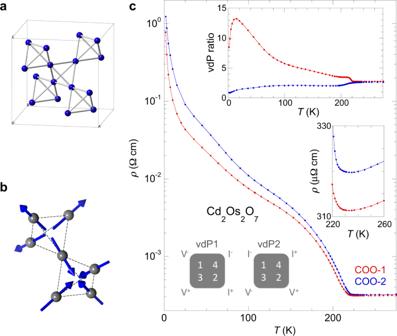Fig. 1: Transport signatures of Cd2Os2O7at zero field. aSchematic of the Os sublattice in the cubic pyrochlore oxide Cd2Os2O7, with all Os atoms forming a three-dimensional corner-sharing octahedra network.bSchematic of AIAO spin arrangement on two adjacent octahedral. Note that this spin arrangement does not break the underlying lattice symmetry.cResistivityρ(T) of Cd2Os2O7measured over two single crystals (COO-1 in red and COO-2 in blue) using the vdP configuration (Schematics). At each temperature, both vdP channels were measured in order to account for the changing current path between the insulating bulk and conductive domain walls. (Top inset) The resistance ratioRvdP2/RvdP1between two vdP channels manifests the changing current path belowTN= 227K. (Bottom inset) Details ofρ(T) nearTN, showing both metallic behavior aboveTN, and also an upturn ofρnear but still aboveTN, which is often attributed to dynamical spin fluctuation effects without long-range order.TNis determined precisely from the magnetic susceptibilityχ(T), individualRvdP2(T) andRvdP1(T) (not shown), andRH(T) in Fig.3a. While Mott insulators induced by Coulomb interactions are a well-recognized class of metal-insulator transitions, insulators purely driven by spin correlations are much less common, as the reduced energy scale often invites competition from other degrees of freedom. Here, we demonstrate a clean example of a spin-correlation-driven metal-insulator transition in the all-in-all-out pyrochlore antiferromagnet Cd 2 Os 2 O 7 , where the lattice symmetry is preserved by the antiferromagnetism. After the antisymmetric linear magnetoresistance from conductive, ferromagnetic domain walls is removed experimentally, the bulk Hall coefficient reveals four Fermi surfaces of both electron and hole types, sequentially departing the Fermi level with decreasing temperature below the Néel temperature, T N = 227 K. In Cd 2 Os 2 O 7 , the charge gap of a continuous metal-insulator transition opens only at T ~ 10 K << T N . The insulating mechanism parallels the Slater picture, but without a folded Brillouin zone, and contrasts sharply with Mott insulators and spin density waves, where the electronic gap opens above and at T N , respectively. Unlike insulators or semiconductors derived from simple metals such as sodium and lithium [1] , [2] , metal-insulator transitions in correlated-electron systems reside outside the paradigm of the single-electron band structure. Factors such as reduced dimensionality and randomness [3] , [4] enrich the description of the critical behavior, with possible separation of spin and charge, and deep connections to exotic states such as high T c superconductivity and quantum spin liquids [5] . In the limit of large electronic correlations, the starting point for discussion is usually the opening of the Hubbard gap [6] , with antiferromagnetic order being a subsidiary effect. There exist several major experimental challenges in establishing a convincing example of a metal-insulator transition driven by spin correlations [7] . First, the spin-correlation energy is typically much smaller than the direct Coulomb interaction, often at a scale comparable to that of the structural modifications induced by the antiferromagnetic order through magnetostrictive effects and symmetry changes, leading to a chicken-and-egg conundrum between ascribing the insulating transition to the lattice and the magnetism [8] , [9] . It is thus preferable to search for candidate systems in which the magnetism would preserve the crystalline symmetry. Materials that demonstrate an all-in−all-out (AIAO) antiferromagnetic order on a pyrochlore lattice, with all four spins on the corner of a tetrahedron pointing either towards or away from the center (Fig. 1 a , b ), meet this criterion. The AIAO order induces no symmetry-breaking magnetostriction and causes an isotropic expansion of the cubic unit cell by a minimal Δ a / a ~ 10 −4 , only becoming experimentally resolvable when T N drops below 40 K [10] , [11] . For AIAO order with T N > 100 K, this overall magnetostriction is fully camouflaged by the thermal lattice contraction [10] , which broadens the bandwidths but introduces no band splitting. The family of AIAO antiferromagnets thus provides a highly desirable model system to investigate spin correlations with little lattice interference. Fig. 1: Transport signatures of Cd 2 Os 2 O 7 at zero field. a Schematic of the Os sublattice in the cubic pyrochlore oxide Cd 2 Os 2 O 7 , with all Os atoms forming a three-dimensional corner-sharing octahedra network. b Schematic of AIAO spin arrangement on two adjacent octahedral. Note that this spin arrangement does not break the underlying lattice symmetry. c Resistivity ρ ( T ) of Cd 2 Os 2 O 7 measured over two single crystals (COO-1 in red and COO-2 in blue) using the vdP configuration (Schematics). At each temperature, both vdP channels were measured in order to account for the changing current path between the insulating bulk and conductive domain walls. (Top inset) The resistance ratio R vdP2 / R vdP1 between two vdP channels manifests the changing current path below T N = 227K. (Bottom inset) Details of ρ ( T ) near T N , showing both metallic behavior above T N , and also an upturn of ρ near but still above T N , which is often attributed to dynamical spin fluctuation effects without long-range order. T N is determined precisely from the magnetic susceptibility χ ( T ), individual R vdP2 ( T ) and R vdP1 ( T ) (not shown), and R H ( T ) in Fig. 3a . Full size image Identifying an AIAO system with a metal-insulator transition represents the next experimental challenge. Accompanying the AIAO order, many 5 d oxides, such as R 2 Ir 2 O 7 ( R = Eu, Sm, and Nd) and Cd 2 Os 2 O 7 (ref. [12] and references in Refs. [11] , [13] , [14] ), also demonstrate a change of temperature dependence in the resistivity at T ~ T N [9] , [13] , [15] , [16] . However, the resistive behavior of R 2 Ir 2 O 7 ( R = Nd, Sm, Eu), especially in the paramagnetic phase, is often inconsistent and raises concerns about their intrinsic, disorder-free behavior [13] , [17] , [18] . Cd 2 Os 2 O 7 has presented consistent behavior in both the electron correlation and metal-insulator transition. Samples from several groups [9] , [15] , [16] always demonstrate magnetic ordering at T N = 225–227 K, metallic behavior above T N , and a three-to-four-decade rise of the resistivity for T < T N in the best samples. This repeatability from crystal to crystal likely indicates a low level of disorder because of the 2+/5+ valence condition of Cd and Os ions as well as the chemical transport growth procedure at low temperature [9] , [15] , [16] . There exists an additional challenge arising from complications in modeling and understanding the transport data in many 5 d AIAO antiferromagnets due to the intrinsically conductive and highly coercive ferromagnetic domain walls [9] , [19] , [20] , [21] . Ferromagnetic domain walls introduce a Zeeman shift in the metallic paramagnetic band structure, but they are not expected to gap the Fermi surface like the antiferromagnetic bulk, and they are expected to remain metallic down to T = 0. As was pointed out recently [21] , the highly coercive metallic ferromagnetic domain walls generate antisymmetric linear magnetoresistance (MR) of the same functional form as the Hall resistance. Moreover, the antisymmetric linear MR is detectable in Hall channels due to the distorted current paths through the domain walls [21] . This effect is likely the root cause of the widely varying Hall coefficient reported in the literature for Cd 2 Os 2 O 7 [9] , [16] , as the standard procedure for extracting Hall resistance through antisymmetrization with respect to magnetic field direction leads to erroneous results. Here we present high-fidelity resistivity and Hall coefficient measurements on single-crystal Cd 2 Os 2 O 7 after employing an intricate procedure to eliminate the influence of conductive ferromagnetic domain walls. Unlike the common understanding of a concurrent metal-insulator transition with the AIAO magnetic transition at T N , our results reveal that Cd 2 Os 2 O 7 is metallic for a broad temperature range below T N , despite an increasing resistivity with decreasing T . It only becomes an insulator at T MIT ~ 10 K, when four sets of Fermi surfaces have sequentially left the Fermi level to open a true electronic gap. This large separation in temperature for spin order ( T N ) and the charge gap ( T MIT ), with T N >> T MIT , unambiguously establishes spin ordering as the driving force in Cd 2 Os 2 O 7 ’s metal-insulator transition. Our methodology in separating the Hall behavior of the bulk from the influences of the domain walls should provide a generic approach to parsing spin and charge effects in correlated antiferromagnetic insulators with metallic domain walls. Insulating behavior at zero field Our single-crystal Cd 2 Os 2 O 7 samples demonstrate a monotonic rise of resistivity over three decades (~3000×) from T N to 1.8 K at zero field (Fig. 1c ), consistent with the best samples reported in the literature [9] , [15] , [16] . Instead of using bar-shaped samples for both resistivity and Hall measurements, our key approach is to utilize the van der Pauw (vdP) configuration of electrical lead placement on plate-shaped samples (ref. [22] , schematics in Figs. 1 c , 2c ). This choice of putting four leads on an equal footing aims to comprehensively evaluate the effects of the electrical current paths, which constantly redistribute between the conductive domain walls and an increasingly insulating bulk as the temperature decreases. As demonstrated by our samples, the vdP ratio, defined as R vdP2 / R vdP1 at zero field, stays constant only in the paramagnetic phase above T N . Below T N , the vdP ratios of two samples have a strong temperature dependence (Fig. 1c , inset) but still evolve continuously as expected from the lack of lattice symmetry breaking in Cd 2 Os 2 O 7 . The resistivity in Fig. 1c is calculated from R vdP2 and R vdP1 at each T according to the standard vdP procedure [22] , an issue we will revisit below. Fig. 2: Separating the influence of metallic ferromagnetic domain walls. a , b Schematics of the measurement procedure using the two-rotator setup. Every galvanomagnetic Cd 2 Os 2 O 7 sample (gray plate) is field-cooled in two stages: a field H is aligned parallel to the sample surface at room temperature before cooling down through T N , and b the sample is rotated below T N to have a field perpendicular to its surface for galvanomagnetic measurements. The in-plane magnetizing direction is defined by angle ϕ at 24 discrete positions, set outside the cryostat at room temperature. c Typical raw data of Hall resistances R ( H ) between two reciprocal channels, measured for sample COO-2 at a specified temperature and magnetization angle ϕ . The difference in slopes indicates the influence of asymmetric linear magnetoresistance from ferromagnetic domain walls [21] . (inset) vdP configuration for the two reciprocal Hall channels. d–f ϕ -dependence of Hall resistivity slopes R H in two reciprocal channels (red and blue) and their average (fresh green), in addition to the resistivity ρ (green) and vdP ratio (orange), measured in sample COO-2 at three temperatures 195, 30, and 1.8 K. (Methods) ( g ) Hall resistivity slopes R H from two reciprocal channels (red and blue) are plotted alongside their average (fresh green) for two different single-crystal Cd 2 Os 2 O 7 samples COO-1 and COO-2. Although the resistance slopes of an individual Hall channel are very different for each sample, with occasional crossings at various temperatures, the averages are similar in shape between the two samples and determine the bulk Hall coefficient R H ( T ). This irregular behavior of resistance slopes of individual Hall channels highlights potential experimental deficiencies in previous Hall measurements. All statistical uncertainties are smaller than the symbols. Full size image Extracting the bulk Hall coefficient The highly coercive, field-independent magnetization M of the conductive ferromagnetic domain walls necessarily introduces antisymmetric linear MR [21] that makes the Hall resistances of the two reciprocal channels, R 12,34 ( H , M ) and R 43,12 ( H , M ), have different linear slopes with H (Fig. 2c ). Due to the cubic symmetry of AIAO order, it is not possible to create a single antiferromagnetic domain and remove the domain walls altogether by field cooling. The separation of galvanomagnetic responses of the bulk domains and the domain walls is instead carried out by introducing a variable M ( ϕ ) through field-cooling along 24 angular directions ϕ within the sample surface plane (Fig. 2 a , b , Methods, and ref. [21] ). Here we first examine the ϕ -dependences of the Hall resistivity slopes from two reciprocal channels \({R}_{{\mathrm{H}}}^{{\mathrm{Hall}}1}\left(\phi \right)\) and \({R}_{{\mathrm{H}}}^{{{\mathrm{Hall}}}2}\left(\phi \right)\) , the vdP ratio, and resistivity ρ ( H = 0), at temperatures 195, 30, and 1.8 K (Fig. 2 d – f ), where the ferromagnetic domain walls have different levels of influence as gauged by the conductance and the bulk Hall coefficient. At all three temperatures (Fig. 2 d − f ), the average slopes of the two Hall resistivities, \({R}_{{\mathrm{H}}}(\phi )=[{R}_{{\mathrm{H}}}^{{{\mathrm{Hall}}}1}\left(\phi \right)+{R}_{{\mathrm{H}}}^{{{\mathrm{Hall}}}2}\left(\phi \right)]/2\) , follow a constraint that (1) \({R}_{{\mathrm{H}}}(\phi )\) are always ϕ -independent. On the other hand, the resultant ϕ -dependent Hall resistivity slopes of the reciprocal channels, \({\Delta R}_{{\mathrm{H}}}^{{{\mathrm{Hall}}}{\mathrm{1,2}}}\left(\phi \right)={R}_{{\mathrm{H}}}^{{{\mathrm{Hall}}}{\mathrm{1,2}}}\left(\phi \right)-{R}_{{\mathrm{H}}}(\phi )\) , behave differently. At 195 and 30 K, \({\Delta R}_{{\mathrm{H}}}^{{{\mathrm{Hall}}}1}\left(\phi \right)\) and \({\Delta R}_{{\mathrm{H}}}^{{{\mathrm{Hall}}}2}\left(\phi \right)\) follow a second constraint that (2) they are identical at ϕ and ϕ + π respectively \({\Delta R}_{{\mathrm{H}}}^{{{\mathrm{Hall}}}1}\left(\phi \right)={\Delta R}_{{\mathrm{H}}}^{{{\mathrm{Hall}}}2}\left(\phi +\pi \right)\) , leading to identical ϕ -averaged resistivity slopes of both Hall channels. From the previous analysis [21] , constraint (1) reflects the voltage−current reciprocity, while constraint (2) manifests Onsager’s reciprocity relation with regard to the ferromagnetic domain wall M . At 1.8 K, the ϕ -dependent Hall resistivity slopes \({\Delta R}_{{\mathrm{H}}}^{{{\mathrm{Hall}}}1}\left(\phi \right)\) and \({\Delta R}_{{\mathrm{H}}}^{{{\mathrm{Hall}}}2}\left(\phi \right)\) (Fig. 2f ) behave differently. Only constraint (1) is sustained, while constraint (2) cannot be satisfied by any choice of the ϕ -independent components. The result is that the ϕ -averaged resistivity slopes of individual Hall channels are no longer necessarily equal to each other and to the ϕ -independent component \({R}_{{\mathrm{H}}}(\phi )\) . The breakdown of constraint (2) seemingly implies a violation of Onsager’s reciprocity relation between ϕ and ϕ + π states. However, the established Onsager’s reciprocity in our system hinges on the inverse relationship between domain wall magnetizations M ( ϕ ) and M ( ϕ + π) through separate field-cooling processes at ϕ and ϕ + π. Their inverse relationship is generally robust in that both ρ and the vdP ratio at zero field demonstrate a π-periodicity at all temperatures (Fig. 2 d – f ). At 1.8 K, the conduction patterns at ϕ and ϕ + π are similar enough to be reproducibly differentiated from those at neighboring ϕ positions, judging by ρ and the vdP ratio (Fig. 2f ). Nevertheless, because of the separate cooldowns, there exist differences beyond an inversion between M ( ϕ ) and M ( ϕ + π). With the increasingly insulating bulk, the electrical current is more concentrated along a fraction of the domain walls, as reflected by the dramatically oscillating vdP ratio from 3:1 to 1:4 (Fig. 2f ). While the entire sample volume brings better averaged galvanomagnetic behavior and demonstrates Onsager reciprocity (Fig. 2 d , e ), probing only a small number of domain walls enhances the relative difference between M ( ϕ ) and M ( ϕ + π). Even at a fixed ϕ , multiple field-coolings can lead to a significant difference in individual Hall channels at 1.8 K (Fig. 2f ), despite the consistency at 30 K (Fig. 2e ). We note that the assumed uniform medium for the vdP technique [22] is justified a posteriori at 195 K and 30 K, as the calculated ρ ( ϕ ) varies within ±0.1% and ±3%, respectively. Constraint (2) remains satisfied (Fig. 2 d , e ). At 1.8 K, ρ ( ϕ ) calculated from the vdP formula [22] varies by ±50% (Fig. 2f ). Although the uniformity assumption no longer holds at 1.8 K to legitimize both the vdP-derived resistivity and constraint (2), our procedure to extract the Hall coefficient R H through the average slope of two Hall resistivity channels is protected by the fundamental principle of voltage−current reciprocity. With the understanding of how to extract R H through a ϕ -dependence study at three fixed temperatures, we now explore the temperature evolution of R H by taking the average Hall resistivity slope of two reciprocal channels at a fixed ϕ (Fig. 2g ). The R H ( T ) measured on two different Cd 2 Os 2 O 7 single crystals (Fig. 3a ) demonstrates a consistent picture that represents the major finding of this work. R H ( T ) remains stable above T N = 227 K, and all bands only start to evolve at T N , maintaining a delicate balance between them until the first sharp change at 220 K. Despite a rise of nearly three orders of magnitude in ρ ( T ) from T N down to 10 K, R H ( T ) remains finite and oscillates between positive and negative values. As ρ ( T ) reflects a fast drop in total carrier density with decreasing temperature (Fig. 1c ), the oscillating R H ( T ) reflects the changes in the bands, with an alternating dominance by either electrons or holes as the major composition of itinerant carriers. In a multiband model with both electron and hole types of carriers, \({R}_{{\mathrm{H}}}\,=\,\tfrac{1}{{ec}}({\sum }_{i\in {\{h\}}}{N}_{i}{\mu }_{i}^{2}\,-\,{\sum }_{j\in {\{e\}}}{N}_{j}{\mu }_{j}^{2})/{({\sum }_{i\in {\{h\}}}{N}_{i}{\mu }_{i}\,+\,{\sum }_{j\in {\{e\}}}{N}_{j}{\mu }_{j})}^{2}\) , with carrier densities \({N}_{i,j}\) and mobilities \({\mu }_{i,j}=e{\tau }_{i,j}/{m}_{i,j}\) determined by the carrier relaxation times \({\tau }_{i,j}\) and masses \({m}_{i,j}\) of individual band i (of holes) or j (of electrons), respectively (Eq. 2.78 of ref. [23] with multiple bands). Here, carrier mobilities are expected to have only a weak temperature dependence. On the other hand, when a band moves out from the Fermi level, the relative contributions of charge carriers (electron or hole) dramatically change, signaled by a rapid turn (over a temperature range ~20 K) in the trend followed by R H ( T ) and similar to other band-gap-opening scenarios exhibited, for example, by charge and spin density waves [24] , [25] . The first surface moves out from the Fermi level at ~220 K (Fig. 3a , top inset), and with R H ( T ) turning more electron-like, the departed carriers are of hole type. As thermal excitation at finite temperature still populates the departed bands close to the Fermi level, R H ( T ) remains a smooth function of T . Here we count four characteristic temperatures below T N —at 220, 165, 80, and 10 K—that reflect four sets of carriers leaving the Fermi level (arrows and T 1 − T 4 in Fig. 3a insets). Below T ~ 10 K, a sharply divergent R H indicates that a full gap emerges in the bulk, and all itinerant carriers are due to thermal excitation, predominately of electron type from the last departed band. Fig. 3: Metal−insulator transition in Cd 2 Os 2 O 7 revealed through bulk Hall coefficient. a Temperature evolution of the bulk Hall coefficient R H ( T ) from two Cd 2 Os 2 O 7 samples COO-1 and COO-2 in Fig. 2g are compared in detail. While R H ( T ) evolves slowly above T N , it starts to deviate from the high-temperature behavior right at T N , indicating that the onset of AIAO antiferromagnetic order influences the band structure around the Fermi level. Nevertheless, R H ( T ) does not diverge until it reaches a temperature below 10 K ~ 0.044 T N when the true charge gap opens. In between, each sharp change in R H ( T ) (close-up view of the main figure in individual insets) indicates a band leaving the Fermi level, marked by arrows at four different temperatures, T 1 = 220 K, T 2 = 165 K, T 3 = 80 K, and T 4 = 10 K. Two bands are of hole type and the other two of electron type. All statistical uncertainties are smaller than the symbols. b Band structure of Cd 2 Os 2 O 7 near the Fermi level. \((E-{E}_{{\mathrm{F}}})\) along trajectories between reciprocal space points \(\Gamma\) , X, W, and L are adapted from calculations in ref. [26] . The four bands, two of hole (green) and two of electron (purple) types, are sequentially driven away from the Fermi level by the increasing strength of antiferromagnetic order to form a band insulator. Full size image Our results can be compared with existing band structure calculations [26] , adapted here in Fig. 3b , that suggest the Fermi surface is made up of three sets of carriers in the paramagnetic phase of Cd 2 Os 2 O 7 : hole surfaces around the W point, an electron shell at the Γ point, and a family of electron ellipsoids along the Γ−X line, solely of Os 5 d t 2g origin. Our observation reveals a fourth set of hole ellipsoids, potentially located along the Γ−X line [26] (Fig. 3b ), but which have an energy difference too small to be resolved by the band structure calculation given that they drop below the Fermi level at 220 K, only 7 K below T N . Infrared reflectivity also illuminates the metal-insulator transition in Cd 2 Os 2 O 7 [27] , [28] . While the direct optical gap has been consistently verified, the interpretation varies from either a spin-density-wave gap opening at T N [27] or an indirect gap opening at ~210 K because of a Liftshitz type of mechanism [28] . The latter is partially consistent with our observed first set of carriers departing the Fermi level at 220 K. Our results demonstrate that the transition at T N = 227 K in Cd 2 Os 2 O 7 should be regarded as only the magnetic-ordering transition, and there is no concurrent metal-insulator transition despite the fact that the resistivity ρ ( T ) changes its temperature dependence around T N (Fig. 1c inset). Given the well-defined changes observed for R H ( T ) at T N (Fig. 3a ), the driving mechanism behind the electronic evolution should be attributed to Os 5 d t 2g band renormalization by the AIAO order [7] , with the effect growing with the increasing strength of the magnetic order parameter, the staggered moment < m >, with decreasing T . From a direct X-ray magnetic diffraction study [12] , < m > continues to grow to the zero-temperature limit without saturation. This spin-dependent shift of the quasiparticles’ self-energy happens within the antiferromagnetic phase and the electronic gap is opened by the developed antiferromagnetic order. It is analogous to a Slater mechanism without Brillouin zone-folding [7] . The entire density of states within ±1.5 eV of the Fermi level is made of the Os 5 d t 2g manifold of 12 bands in total (two Cd 2 Os 2 O 7 units in the primitive unit cell, with three t 2g bands from individual Os ions) [26] . Due to the Os 5+ (5 d 3 ) valence, these bands are filled between the sixth and seventh bands, with dispersion across the Fermi surface to create the electron-type and hole-type carriers. Spin correlation renormalizes the t 2g manifold to create a true gap at the half level between the sixth and seventh bands. The Mott−Hubbard picture of the metal-insulator transition splits a single band to open a gap by strong charge correlation energy ( U ~ 2−6 eV). In Cd 2 Os 2 O 7 , an AIAO antiferromagnet with no structural instability, the transition relies on a small spin-correlation energy ( T N ~ 20 meV) to essentially create a band insulator. The spin and charge gaps are widely separated in temperature. However, they remain experimentally obscure until the confounding effects of metallic domain wall conduction can be separated from the intrinsic bulk behavior. The methods introduced here clarify the contributions from the bulk and the role of the spin and charge degrees of freedom. They also promise a means to quantify the conductive properties of coercive ferromagnetic domain walls winding their way through an insulating antiferromagnet. Sample origin and preparation In this work, we used high-quality Cd 2 Os 2 O 7 single crystals from ref. [9] ; the vapor transport growth techniques and catalog of physical characteristics are detailed therein. The single crystals used in this work were of octahedral shape and 0.3−0.5 mm in size. Individual crystals were polished to plates of 17−20 μm thickness with a (1, 1, 0) surface normal [14] . Previous synchrotron X-ray magnetic diffraction studies directly verified the quality of these single-crystal plates, demonstrating typical crystal mosaics of 0.01−0.02 o FWHM and the existence of AIAO order [14] . Further, the pyrochlore space group Fd-3m was verified to the highest sensitivity possible by examining the forbidden orders of (4, 2, 0) and (6, 0, 0) using synchrotron-based single-crystal x-ray diffraction [14] . Samples were selected for these transport measurements from unused plates prepared for the X-ray study, which are of better quality than the sample used in a previous galvanomagnetic study [21] . The sample in ref. [21] was cut from a large crystal (3 × 3× 1 mm 3 ) with a significantly broader mosaic (supplementary materials of ref. [21] ), and higher density of domain walls, as indicated by a comparison of Fig. 2d in this work to Fig. 3f of ref. [21] . Galvanomagnetic measurements As the current distribution could potentially change under temperature between the domain walls and bulk, a strict Hall bar-shaped sample geometry is not advantageous, as it could have potentially complex issues in translating from measured resistances to the underlying resistivity. Instead, we employ a van der Pauw (vdP) sample geometry [22] , where the standard conversion depends only on the sample thickness rather than all lateral dimensions. Furthermore, the vdP geometry allows equal access to all combinations of lead configurations in the measurement of both Hall and magnetoresistance (Figs. 1 c and 2c insets) [21] . Four 25 μm diameter gold wires were attached to the transport samples of typical 200 μm lateral sizes by conductive silver epoxy. The transport samples were mounted on the standard sample holder of a horizontal rotator probe in a 14 T Physical Property Measurement System (PPMS, Quantum Design, Inc.). Using the horizontal rotation, we first cool our samples through T N with a 2 T magnetic field applied along an in-plane direction ϕ (Fig. 2a ) then the sample is rotated below T N to allow the measurement magnetic field of both the Hall effect and the MR to be applied perpendicular to the sample surface (Fig. 2b ). 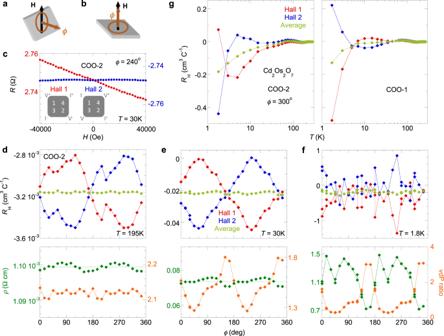Fig. 2: Separating the influence of metallic ferromagnetic domain walls. a,bSchematics of the measurement procedure using the two-rotator setup. Every galvanomagnetic Cd2Os2O7sample (gray plate) is field-cooled in two stages:afieldHis aligned parallel to the sample surface at room temperature before cooling down throughTN, andbthe sample is rotated belowTNto have a field perpendicular to its surface for galvanomagnetic measurements. The in-plane magnetizing direction is defined by angleϕat 24 discrete positions, set outside the cryostat at room temperature.cTypical raw data of Hall resistancesR(H) between two reciprocal channels, measured for sample COO-2 at a specified temperature and magnetization angleϕ. The difference in slopes indicates the influence of asymmetric linear magnetoresistance from ferromagnetic domain walls21. (inset) vdP configuration for the two reciprocal Hall channels.d–fϕ-dependence of Hall resistivity slopesRHin two reciprocal channels (red and blue) and their average (fresh green), in addition to the resistivityρ(green) and vdP ratio (orange), measured in sample COO-2 at three temperatures 195, 30, and 1.8 K. (Methods) (g) Hall resistivity slopesRHfrom two reciprocal channels (red and blue) are plotted alongside their average (fresh green) for two different single-crystal Cd2Os2O7samples COO-1 and COO-2. Although the resistance slopes of an individual Hall channel are very different for each sample, with occasional crossings at various temperatures, the averages are similar in shape between the two samples and determine the bulk Hall coefficientRH(T). This irregular behavior of resistance slopes of individual Hall channels highlights potential experimental deficiencies in previous Hall measurements. All statistical uncertainties are smaller than the symbols. 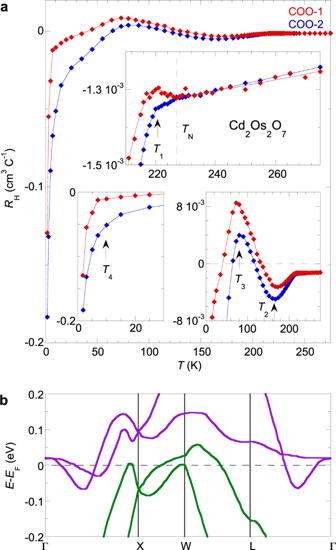Fig. 3: Metal−insulator transition in Cd2Os2O7revealed through bulk Hall coefficient. aTemperature evolution of the bulk Hall coefficientRH(T) from two Cd2Os2O7samples COO-1 and COO-2 in Fig.2gare compared in detail. WhileRH(T) evolves slowly aboveTN, it starts to deviate from the high-temperature behavior right atTN, indicating that the onset of AIAO antiferromagnetic order influences the band structure around the Fermi level. Nevertheless,RH(T) does not diverge until it reaches a temperature below 10 K ~ 0.044TNwhen the true charge gap opens. In between, each sharp change inRH(T) (close-up view of the main figure in individual insets) indicates a band leaving the Fermi level, marked by arrows at four different temperatures,T1= 220 K,T2= 165 K,T3= 80 K, andT4= 10 K. Two bands are of hole type and the other two of electron type. All statistical uncertainties are smaller than the symbols.bBand structure of Cd2Os2O7near the Fermi level.\((E-{E}_{{\mathrm{F}}})\)along trajectories between reciprocal space points\(\Gamma\), X, W, and L are adapted from calculations in ref.26. The four bands, two of hole (green) and two of electron (purple) types, are sequentially driven away from the Fermi level by the increasing strength of antiferromagnetic order to form a band insulator. An additional home-built indexing stage on the sample holder provides degree of freedoms to set field-cooling along 24 discrete angular positions of ϕ within the sample surface plane [21] ; the origin of the ϕ -angle has no specific relationship to either the wiring positions of the electrical leads or the crystalline structure. Galvanomagnetic responses of both reciprocal Hall channels and vdP channels were measured at selected temperatures of 195, 30, and 1.8 K for the full ϕ -dependence (Fig. 2 d − f ). The data set at 195K was measured independently from those at the other two temperatures. At 30 and 1.8 K, measurements were repeated at three and eleven ϕ positions, respectively, for a check of reproducibility through an additional field-cooling process. For measurements at 30 K, all data except two (one each at ϕ = 30 o and 195 o ) have a corresponding measurement at 1.8 K during the same field-cooling process in order to compare the ϕ -dependence at both temperatures. For the full temperature evolution in Figs. 1 , 2g , and 3 , both samples were field-cooled along one in-plane ϕ position to base temperature; then the galvanomagnetic measurements were performed at each stabilized temperature along the warming trajectory. We observe no degrading or change in our samples after many thermal cycles (>60 in COO-2). The resistivity was measured using a Lakeshore LS372 AC resistance bridge, working at 9.8 Hz, together with a low-noise 3708 preamp and a home-built vdP switching box based on low-resistance CMOS relay switches. At zero field, the vdP relationship is satisfied to Δ R / R max = ( R Hall1 + R vdP1 − R vdP2 )/Max( R vdP1 : R vdP2 ) < ±0.05% at 30 K and <±0.25% at 1.8 K. R ( H ) curves were measured over a magnetic field loop of ±4 T The coercive field of the ferromagnetic domain walls is known to be >9 T (see, e.g., ref. [20] ), and our measurements over field loops of ±14 T also demonstrate repeatable field dependence. We thus conclude that the domain wall configuration stays constant during each measurement. Since no field hysteresis was observed, R ( H ) values are averaged at each field, exemplified by Fig. 2c , and fit to a polynomial form to the second order. The linear slope is taken for plots in Figs. 2 and 3 . Our samples demonstrate a very low level of positive parabolic MR ~0.3% over ±14 T, consistent from 1.65 to 80 K, and is thereby unappreciable at low fields. The low level of MR indicates that the cyclotron frequency \({\omega }_{c}\) and carrier relaxation time \(\tau\) satisfy \({\omega }_{c}\tau \ll 1\) , and the measured Hall coefficient R H ( T ) is in the low-field limit.